Inhibition of specific gene expressions by protein-mediated mRNA interference RNA interference mediated by RNA such as antisense RNA, short interfering RNA and micro RNA is well documented to regulate specific gene expression at the level of messenger RNA. However, RNA interference mediated by proteins has not been reported. Here we identify the MazF-hw mRNA interferase from a superhalophilic archaeon that cleaves RNA at a specific seven-base sequence (UUACUCA). This sequence was found unusually abundant in the mRNAs for rhodopsin transcription activator and some membrane proteins of the archaeon, suggesting that the expression of these proteins is regulated by MazF-hw. When all of the seven-base cleavage sites in essential genes in Escherichia coli were eliminated, the cells were no longer sensitive to MazF-hw, demonstrating that specific gene expression can be regulated by a sequence-specific mRNA interferase. These findings demonstrate that mRNA interference can be mediated not only by RNA but also by proteins to effectively silence specific gene expression in cells. RNA-mediated messenger RNA interference has been well documented including the initial finding of a natural antisense RNA in Escherichia coli [1] and its application to regulate specific gene expression [2] and to prevent phage infection [3] . In eukaryotic cells, small antisense RNA molecules such as micro RNA (miRNA) [4] and short interfering RNA (siRNA) [5] , [6] have been also reported. A common mechanism for all these systems is the use of an RNA sequence complementary to a target mRNA to silence the mRNA. Since the original discovery of an ACA-specific mRNA interferase, MazF, in E. coli [7] , a number of MazF homologues have been found in other bacteria, which cleave mRNA at specific three- or five-base sequences (see a review in ref. 8 ). However, the three- or five-base cleavage sequences by these mRNA interferases are too short for silencing the expression of a specific gene or a specific group of genes to regulate cell growth. We have identified a new MazF homologue from Haloquadra walsbyi isolated from a hypersaline pool on the Sinai Peninsula [9] , which cleaves RNA at a specific seven-base sequence. This archaeon is square-shaped but extremely thin; 2–5 μm in width and less than 0.2 μm in thickness [9] , [10] , resembling other super halophilic microorganisms that require 3–4 M NaCl for growth and are tolerant in 2 M magnesium [11] . H. walsbyi grows phototrophically using bacteriorhodopsin in the membrane [12] . Here we demonstrate that the protein, which is homologous to E. coli MazF, has a much higher sequence-specificity cleaving RNA at a specific seven-base RNA sequence, demonstrating for the first time protein-mediated mRNA interference to silence specific gene expression. These results further imply that mRNA interferases may be widely applicable for regulation of specific gene expression to regulate cell growth from bacteria to human. Identification of a MazF homologue in H. walsbyi We performed a blast analysis of the H. walsbyi genome to search for a gene encoding a homologue of the E. coli MazF protein; we identified the gene HQ2202A that encodes a 124-residue protein. This protein has 31% identity and 46% similarity to E. coli MazF consisting of 111 residues ( Fig. 1a ). Notably, there is a gene immediately upstream of the gene for MazF-hw, and they overlap each other by four bases in a similar manner to that of the E. coli mazE–mazF operon [13] ( Fig. 1b ). However, the upstream open reading frame (ORF) (termed MazY-hw) does not show homology to E. coli MazE, the antitoxin of MazF. 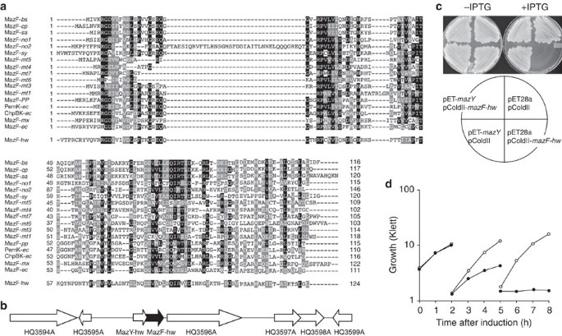Figure 1: MazF homologue fromH. walsbyi. (a) Alignment of MazF-hw with other MazF homologues fromB. subtilis168 (MazF-bs),C. perfigens13 (MazF-cp),S. aureusCOL (MazF-sa),NostocPCC7120 (MazF-no),SynechocystisPCC6803 (MazF-sy),M. tuberculosisH37Rv (MazF-mt1 to -mt7), ChpBK inE. coli(ChpBK-ec), PemK inE. coli(PemK-ec),M. xanthus(MazF-mx) and MazF fromE. coliK12 (MazF-ec). Identical amino acid residues are shown in black shades and conservative substitutions in grey shades. (b) Location of themazF-hwgene on theH. walsbyichromosome obtained from TIGR. (c) Toxicity ofH. walsbyiMazF-hw on M9-glycerol-casamino acids plates with and without IPTG (0.1 mM). (d) Effect of MazF-hw induction on cell growth.E. coliBL21 cells harbouring pColdII-mazF-hwwere cultured in M9-glycerol-casamino acids medium at 37 °C until cell density reached 30 Klett (3×107cells ml−1). Then, the culture was divided into two; one was incubated at 37 °C with (closed circles) and the other without IPTG (0.1 mM; open circles). The cultures were diluted tenfold at 2 h and 5 h time points, respectively, and the cell density was measured for 8 h. Figure 1: MazF homologue from H. walsbyi. ( a ) Alignment of MazF-hw with other MazF homologues from B. subtilis 168 (MazF-bs), C. perfigens 13 (MazF-cp), S. aureus COL (MazF-sa), Nostoc PCC7120 (MazF-no), Synechocystis PCC6803 (MazF-sy), M. tuberculosis H37Rv (MazF-mt1 to -mt7), ChpBK in E. coli (ChpBK-ec), PemK in E. coli (PemK-ec), M. xanthus (MazF-mx) and MazF from E. coli K12 (MazF-ec). Identical amino acid residues are shown in black shades and conservative substitutions in grey shades. ( b ) Location of the mazF-hw gene on the H. walsbyi chromosome obtained from TIGR. ( c ) Toxicity of H. walsbyi MazF-hw on M9-glycerol-casamino acids plates with and without IPTG (0.1 mM). ( d ) Effect of MazF-hw induction on cell growth. E. coli BL21 cells harbouring pColdII- mazF-hw were cultured in M9-glycerol-casamino acids medium at 37 °C until cell density reached 30 Klett (3×10 7 cells ml −1 ). Then, the culture was divided into two; one was incubated at 37 °C with (closed circles) and the other without IPTG (0.1 mM; open circles). The cultures were diluted tenfold at 2 h and 5 h time points, respectively, and the cell density was measured for 8 h. Full size image To examine the MazF-hw toxicity in E. coli , the mazF-hw gene was synthesized and cloned into pColdII vector. As shown in Figure 1c , the induction of MazF-hw inhibited colony formation on an agar plate in the presence of 0.1 mM isopropyl-β- D -1-thiogalactoside (IPTG). We also synthesized the gene for MazY-hw and cloned it into pET28a. As shown in Figure 1c , co-induction of MazY-hw with MazF-hw neutralized the toxicity of MazF-hw, indicating that MazY-hw is the antitoxin for MazF-hw. We also examined the toxicity of MazF-hw in a liquid culture ( Fig. 1d ). When MazF-hw was induced by the addition of 0.1 mM IPTG, cell growth was completely inhibited but only after 5 h or three generations. This slow growth inhibition is in a sharp contrast to that observed with E. coli MazF, which completely inhibits cell growth within 15 min after induction [7] . We speculated that this slow inhibitory effect of MazF-hw was likely due to its RNA cleavage specificity. MazF-hw is an mRNA interferase Next, we purified MazF-hw protein to determine its cleavage specificity. First, we used 3.5-kb MS2 phage RNA as substrate and found that MazF-hw cleaves this RNA only at one site ( Fig. 2a ). The reaction was carried out in the presence of CspA, an RNA chaperone, which prevents the formation of secondary structures in RNA [14] . It is important to note that preincubation of MazF-hw with MazY-hw completely inhibited its endoribonuclease activity, suggesting that the observed cleavage was caused by MazF-hw ( Fig. 2a ; lane 4). The specific cleavage site in MS2 RNA was determined between ---ACUUU and ACUCA--- by primer extension ( Fig. 2b ). We next used 16S and 23S ribosomal RNAs from E. coli and 18S and 28S rRNAs from yeast as substrates. Surprisingly, none of these RNAs were cleaved by MazF-hw ( Fig. 2c,d , respectively). The cleavage activity was completely inhibited by the addition of 10 mM MgCl 2 in the reaction mixture as found with E. coli MazF [7] and required 10–100 mM NaCl ( Fig. 2e ). Using Perl programming language for computational analysis, we analysed these RNAs for all possible four, five and six-base RNA sequences that also include the sequence at the sole cleavage in size found in MS2 RNA, to find sequences present in MS2 RNA but absent in the rRNAs in E. coli and yeast. The results, presented in Table 1 , demonstrate that there are two possible six-base RNA cleavage sequences for MazF-hw, U UACUC and UACUC A, neither of which exists in E. coli 16S and 23S rRNAs and in yeast 18S and 28S rRNAs (the common bases in the sequences are underlined). 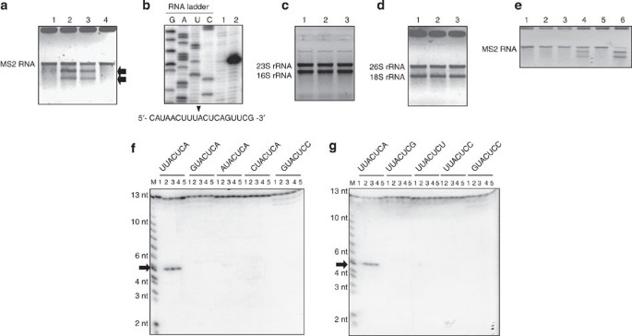Figure 2: Endoribonuclease activity of MazF-hwin vitro. Cleavage of MS2 phage RNA by MazF-hw (a), (b) Analysis of MazF-hw cleavage sites in MS2 phage RNA byin vitroprimer extension. Lane 1 represents a control reaction in which no protein was added; lane 2, MS2 RNA was incubated with MazF-hw. The cleavage site is indicated by an arrow on the RNA sequence and determined using the RNA ladder shown on the bottom. Cleavage ofE. colitotal RNA (c), and yeast total RNA (d) by MazF-hw. Purified MazF-hw was incubated with each substrate at 37 °C for 30 min with (lane 2) or without (lane 3) purified CspA protein20. MazY-hw was mixed with MazF-hw and incubated on ice for 10 min. Then, the mixture was incubated with MS2RNA for 30 min at 37 °C (lane 4). The products are indicated by arrows. (e) Endoribonuclease activity of MazF-hw in the presence of MgCl2and NaCl. Purified MazF-hw was incubated with MS2 phage RNA. The reaction mixture (20 μl) consisted of 0.8 μg MS2 RNA, 0.5 μg MazF-hw and 0.5 μl of RNase inhibitor in 20 mM Tris–HCl (pH8.0) in the absence (lane 1) or in the presence of MgCl2and NaCl (lanes 2–6). Lane 2, 10 mM MgCl2; lane 3, 100 mM MgCl2; lane 4, 10 mM NaCl; lane 5, 400 mM NaCl; lane 6, 100 mM NaCl. Synthesized 13-base RNA (5′- A1A2G3U4U5A6C7U8C9A10A11A12G13-3′) in which the U4 residues were replaced with A, G, and C (f) or A10 residues were replaced with G, C, and U residues (g), respectively, used as substrates. The substrates labelled at the 5′-end with32P were incubated with MazF-hw for 0, 2, 5 and 10 min (lanes 1–4, respectively) or without MazF-hw for 10 min (lane 5). Figure 2: Endoribonuclease activity of MazF-hw in vitro . Cleavage of MS2 phage RNA by MazF-hw ( a ), ( b ) Analysis of MazF-hw cleavage sites in MS2 phage RNA by in vitro primer extension. Lane 1 represents a control reaction in which no protein was added; lane 2, MS2 RNA was incubated with MazF-hw. The cleavage site is indicated by an arrow on the RNA sequence and determined using the RNA ladder shown on the bottom. Cleavage of E. coli total RNA ( c ), and yeast total RNA ( d ) by MazF-hw. Purified MazF-hw was incubated with each substrate at 37 °C for 30 min with (lane 2) or without (lane 3) purified CspA protein [20] . MazY-hw was mixed with MazF-hw and incubated on ice for 10 min. Then, the mixture was incubated with MS2RNA for 30 min at 37 °C (lane 4). The products are indicated by arrows. ( e ) Endoribonuclease activity of MazF-hw in the presence of MgCl 2 and NaCl. Purified MazF-hw was incubated with MS2 phage RNA. The reaction mixture (20 μl) consisted of 0.8 μg MS2 RNA, 0.5 μg MazF-hw and 0.5 μl of RNase inhibitor in 20 mM Tris–HCl (pH8.0) in the absence (lane 1) or in the presence of MgCl 2 and NaCl (lanes 2–6). Lane 2, 10 mM MgCl 2 ; lane 3, 100 mM MgCl 2 ; lane 4, 10 mM NaCl; lane 5, 400 mM NaCl; lane 6, 100 mM NaCl. Synthesized 13-base RNA (5′- A 1 A 2 G 3 U 4 U 5 A 6 C 7 U 8 C 9 A 10 A 11 A 12 G 13 -3′) in which the U4 residues were replaced with A, G, and C ( f ) or A10 residues were replaced with G, C, and U residues ( g ), respectively, used as substrates. The substrates labelled at the 5′-end with 32 P were incubated with MazF-hw for 0, 2, 5 and 10 min (lanes 1–4, respectively) or without MazF-hw for 10 min (lane 5). Full size image Table 1 Speculated MazF-hw cleavage sites for select RNAs. Full size table MazF-hw cleaves RNA at a specific seven-base sequence To determine which of the two sequences was the actual cleavage site, we first synthesized two 13-base oligonucleotides, 5′-AAGU UACUC CAGG-3′ and 5′-AAGC UACUC AAGG-3′. The underlined sequences are from MS2 RNA including the common UACUC sequence. However, neither of the RNAs was cleaved by MazF-hw. Subsequently, we synthesized 7 more 13-base oligoribonucleotides, which have various bases on both sides of the 6-base central common sequences ( Fig. 2f,g ). Surprisingly, MazF-hw cleaved only one of these substrates, UUACUCA, which matches well with the cleavage sequence found in MS2 RNA. The amount of cleaved products of UUACUCG and other RNAs are less than 1% compared with UUACUCA ( Fig. 2f,g ). This feature was not affected by the incubation conditions such as salt concentration and temperature. Thus, we concluded that MazF-hw recognizes the seven-base sequence, UU^ACUCA and cleaves between the second (U) and the third residue (A) (^ indicates the cleavage site). As a specific seven-base sequence can be found on average only once every 16,384-base RNA sequence, we speculated that MazF-hw cleaves only a specific group of mRNAs in H. walsbyi . Out of 2,610 ORFs on the H. walsbyi genome, only 183 ORFs have the seven-base sequence, of which one has three seven-base sequences, twelve have two ( Table 2 ), and the remaining 170 ORFs have only one ( Supplementary Data 1 ). As one can assume that the mRNA sensitivity to MazF-hw is proportional to the number of the seven-base cleavage sites present, the boa gene for a putative transcription activator for rhodopsin (bacterio-opsin) having three seven-base sequences may be the most sensitive, suggesting that, on induction of MazF-hw, the expression of the light-driven proton pump may be turned off. Table 2 The most MazF-hw sensitive ORFs in H. walsbyi. Full size table Regulation of specific gene by MazF-hw in E. coli In E. coli , out of 233 ORFs containing the 7-base sequence, only 4 ( lolD, rplC, rpmD and rpoB ,) are essential for cell growth ( Supplementary Data 2 ). On MazF-hw induction, mRNAs from all four of these genes were degraded ( Fig. 3a,b ). However, the ompA mRNA, which does not contain UUACUCA sequences was stable after induction of MazF-hw, indicating that MazF-hw cleaves only at UUACUCA sequence ( Fig. 3c ). We then tested whether MazF-hw was no longer toxic to E. coli , if all the cleavage sites in these four genes were altered to non-MazF-hw cleavage sites. 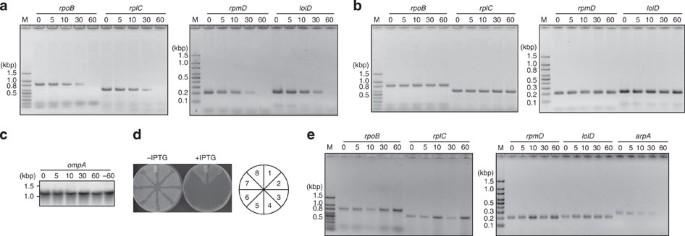Figure 3: Four essential genes containing hepta-sequence are essential for MazF-hw toxicity. Total RNA was extracted fromE. coliBL21(DE3) cells harbouring pColdII-mazF-hw(a) and pColdII (b) at various time points after the addition of 0.1 mM IPTG and subjected to reverse transcriptase PCR (RT–PCR). (c) Effect of MazF-hw onompAmRNA. Northern blot analysis was carried out with total RNA described above. The probe was prepared using High Prime (Roche) following the manufacturer's protocol. (d) The UUACUCA-lessrpoBandlolDgenes were cloned into pACYCDuet, and UUACUCA-lessrplCandrpmDgenes were cloned into pCOLADuet.E. coliBL21 (DE3) cells harbouring both of these plasmids and pColdII-mazF-hw (1 to 8). These cells contain plasmids as follows: 1, pACYCDuet, pCOLADuet and pColdII; 2, pACYCDuet, pCOLADuet and pColdII-mazF-hw; 3, pACYC-lolD, pCOLA-rplC-rpmDand pColdII-mazF-hw; 4, pACYC-rpoB-lolD, pCOLA-rpmDand pColdII-mazF-hw; 5, pACYC-rpoB-lolD, pCOLA-rplCand pColdII-mazF-hw; 6, pACYC-rpoB, pCOLA-rplC-rpmDand pColdII-mazF-hw; 7, pACYC-rpoB*-lolD*, pCOLA-rplC*-rpmD*and pColdII-mazF-hw; and 8, pACYC-rpoB-lolD, pCOLA-rplC-rpmDand pColdII-mazF-hw(asterisk means the genes contain UUACUCA sequence) were streaked on M9 plates with or without 0.1 mM IPTG and incubated at 30 °C for 20 h. All the three vectors were used as controls. (e) Total RNA was extracted fromE. coliBL21(DE3) cells harbouring pColdIImazF-hwand UUACUCA-less four genes at various time points after the addition of 0.1 mM IPTG and subjected to RT–PCR. As shown in Figure 3d , cell growth was not sensitive to MazF-hw induction. However, cell growth was sensitive to MazF-hw, when the four genes contain a UUACUCA sequence ( Fig. 3d ). Notably, even when one of the four genes was left intact, cell growth was blocked on induction of MazF-hw, in the presence of IPTG. Although mRNAs from all four of these genes were resistant to MazF-hw, the arpA mRNA containing UUACUCA sequences was degraded in the cells ( Fig. 3e ). These data demonstrate that specific genes can be silenced by a sequence-specific mRNA interferase. These data also confirmed that MazF-hw cleaves mRNA specifically at the UUACUCA sequences. Figure 3: Four essential genes containing hepta-sequence are essential for MazF-hw toxicity. Total RNA was extracted from E. coli BL21(DE3) cells harbouring pColdII- mazF-hw ( a ) and pColdII ( b ) at various time points after the addition of 0.1 mM IPTG and subjected to reverse transcriptase PCR (RT–PCR). ( c ) Effect of MazF-hw on ompA mRNA. Northern blot analysis was carried out with total RNA described above. The probe was prepared using High Prime (Roche) following the manufacturer's protocol. ( d ) The UUACUCA-less rpoB and lolD genes were cloned into pACYCDuet, and UUACUCA-less rplC and rpmD genes were cloned into pCOLADuet. E. coli BL21 (DE3) cells harbouring both of these plasmids and pColdII- mazF -hw (1 to 8). These cells contain plasmids as follows: 1, pACYCDuet, pCOLADuet and pColdII; 2, pACYCDuet, pCOLADuet and pColdII- mazF-hw ; 3, pACYC- lolD , pCOLA- rplC-rpmD and pColdII- mazF-hw ; 4, pACYC- rpoB - lolD , pCOLA -rpmD and pColdII- mazF-hw ; 5, pACYC- rpoB - lolD , pCOLA- rplC and pColdII- mazF-hw ; 6, pACYC- rpoB , pCOLA- rplC-rpmD and pColdII- mazF-hw ; 7, pACYC- rpoB* - lolD* , pCOLA- rplC*-rpmD* and pColdII- mazF-hw ; and 8, pACYC- rpoB - lolD , pCOLA- rplC-rpmD and pColdII- mazF-hw (asterisk means the genes contain UUACUCA sequence) were streaked on M9 plates with or without 0.1 mM IPTG and incubated at 30 °C for 20 h. All the three vectors were used as controls. ( e ) Total RNA was extracted from E. coli BL21(DE3) cells harbouring pColdII mazF-hw and UUACUCA-less four genes at various time points after the addition of 0.1 mM IPTG and subjected to RT–PCR. Full size image In this report, we demonstrate that H. walsbyi contains a MazF homologue, which is a seven-base (UUACUCA)-specific mRNA interferase. Such a highly sequence-specific mRNA interferase may be called an RNA restriction enzyme, as DNA restriction enzymes are also specific to certain DNA sequences for their cleavage. Notably, however, since DNA restriction enzymes require a palindromic sequence at the cleavage sites, there are only 64 different sequences in the six-base sequences. On the other hand, mRNA interferases recognize a single-stranded RNA, and there are 4,096 possible sequences for the 6-base sequences and 16,384 possible sequences for the 7-base sequences. Out of all 2,610 ORFs on the H. walsbyi genome (NCBI RefSeq accession number Accession NC_008212 ), only 183 ORFs contain at least one UUACUCA sequence ( Supplementary Data 1 ). Of these 183 genes, one gene, boa , encoding a transcriptional regulator for rhodopsin, contains three of the seven-base sequence, suggesting that the light-driven proton pump is effectively regulated at the level of mRNA by an mRNA interferase. It has been shown that E. coli MazF causes complete cell growth arrest, however the cells retain full metabolic activity [7] . This physiological quasi-dormant state caused by MazF induction is considered to play an important role in cellular survival under various stress conditions in nature. Notably, the MazF-hw activity was strongly inhibited in the presence of 10 mM MgCl 2 or 400 mM NaCl ( Fig. 2e ), while H. walsbyi requires 3 M NaCl for growth and is resistant to 2 M MgCl 2 (refs 11 , 12 ), suggesting that MazF-hw is likely not to be active under normal growth conditions in nature. This archaeon lives floating on the surface of saturated salt water [9] , thus effectively utilizing sun light for the production of ATP. However, it is assumed that on hypo-osmotic stress such as rain fall or the influx of water from a river the specific gravity of the saturated salt water is lower, the cells can no longer float on the surface, resulting in a reduction in ATP production. As a result, the cellular salt concentration decreases causing the activation of MazF-hw, which then degrades the mRNA for the transcription activator for the rhodopsin gene. Most of the genes containing two of the seven-base sequence such as ABC-type transporters, cAMP-dependent carbon starvation protein A, sulfatase and FAD-linked oxidase ( Table 2 ) also seem to be involved in hypo-osmotic stress. While sequence-specific DNA restriction enzymes have been known for many years, mRNA interferases have only recently been discovered [8] , [15] , [16] . To date, a number of MazF homologues are found in bacteria, having a wide range of cleavage specificities from three to five bases. It has been shown that pathogenic bacteria such as Mycobacterium tuberculosis [14] , [17] and Staphylococcus aureus [18] contain mRNA interferases that recognize specific five-base RNA sequences, which are either overpresented or underpresented in genes associated with their pathogenicity. In Myxococcus xanthus , a five-base sequence-specific mRNA interferase has been show to be required for programmed cell death during fruiting body formation [19] . These five-base specific mRNA interferases may be sufficient to silence a group of genes sharing cellular functions such as pathogenecity and cellar development, but specific enough to target only a single gene or only a few limited target genes. To achieve protein-mediated mRNA interference comparable to RNA-mediated mRNA interference, much higher sequence-specific mRNA interferases are required. The present discovery of MazF-hw, specific to a seven-base RNA sequence, raises an intriguingly possibility that there may be many other MazF homologues for other seven-base or longer RNA sequences so that only a specific mRNA or a specific group of cellular mRNAs can be silenced using the highly specific mRNA interferases. One may also engineer novel mRNA interferases having different cleavage specificities on the basis of known MazF homologues. Although the seven-base cutter, MazF-hw, is not specific enough to regulate expression of specific human genes ( Supplementary Data 3 ), it is possible to engineer MazF-hw to be more specific targeting only a few human genes. The structural study of the mRNA interferase-RNA complex may provide important clues for designing of more highly sequence-specific mRNA interferases to regulate specific human gene expression. Notably, in addition to antisense RNA and siRNA technology, protein-mediated RNA interference with the use of mRNA interferases will open up a new avenue to interfere with the expression of a specific mRNA or a specific group of mRNAs, preventing viral infection and harmful gene expression from bacteria to human. Bacterial strains and plasmids E. coli BL21(DE3) and DH5α were used. The mazF-hw gene was synthesized (Genscript) and cloned into pColdII (Takara Bio) to express the MazF-hw. The four genes ( rpoB, lolD, rplC and rpmD ) were amplified by PCR using the E. coli genomic DNA as template and primers ( Supplementary Table S1 ) and then cloned into pACYCDuet and pCOLADuet (Novagen), respectively. Site-directed mutagenesis was carried out with Primestar polymerase (Takara Bio). Protein purification To purify N-terminal His-tagged MazF-hw, pColdII– mazF-hw was introduced into E. coli BL21(DE3). The expression of MazF-hw was induced with 1 mM isopropyl-β- D -1-thiogalactoside (IPTG) at 15 °C for 3 h. The MazF-hw was purified with Ni-NTA agarose (Qiagen) following the manufacturer's protocol. mRNA interferase activity of MazF-hw Purified MazF-hw was incubated with E. coli total RNA, yeast total RNA and MS2 phage RNA at 37 °C for 30 min with or without purified CspA protein, an RNA chaperone [20] . The reaction mixture (20 μl) consisted of each RNA, 0.5 μg MazF-hw, 120 μg CspA, 0.1 mM EDTA, 100 mM NaCl and 0.5 μl of RNase inhibitor (Roche) in 20 mM Tris–HCl (pH 8.0). After denaturation in urea, the products were separated on a 1.2% agarose gel [14] , [21] . Primer extension analysis in vitro MS2 RNA was incubated with or without purified MazF-hw, as described above. Primer extension was carried out at 47 °C for 1 h with 10 units of AMV-reverse transcriptase (AMV-RT) (Roche) with the 0.8 μg of MS2 RNA and 1 pmol of the primer ( Supplementary Table S1 ) labelled with [ γ - 32 P]–ATP. The reaction was stopped by the addition of sequencing loading buffer (95% formamide, 20 mM EDTA, 0.05% bromophenol blue and 0.05% xylene cyanol) and heated at 95 °C for 2 min and then placed on ice. The products were analysed on a 6% polyacrylamide containing 8 M urea gel with a sequencing ladder made with same primer [21] . Cleavage of synthetic RNA by MazF-hw Synthesized 13-base RNA (5′-A 1 A 2 G 3 U 4 U 5 A 6 C 7 U 8 C 9 A 10 A 11 A 12 G 13 -3′) in which the U4 and A10 residues were replaced with A, G, and C or G, C, and U residues, respectively, were used as substrate. The labelled substrates with [ γ - 32 P]–ATP using T4 kinase (New England Biolabs) were incubated with MazF-hw for 0, 5 and 30 min or without MazF-hw for 30 min at 20 °C in a reaction mixture containing 20 mM Tris–HCl (pH 8.0), 1 mM EDTA, 100 mM NaCl and 0.5 μl of RNase inhibitor. To analyse synthetic RNA cleavage, the products were analysed on a 20% polyacrylamide gel containing 8 M urea with a ladder [22] . Northern blotting analysis of ompA mRNA E. coli cells containing pColdII- mazF-hw were grown at 37 °C in M9-glucose. When the O.D. 600 value reached 0.4, IPTG was added to a final concentration of 1 mM. The samples were taken at different intervals. Total RNA was extracted using hot phenol method [21] . Samples containing 2 μg of RNA were loaded onto a 1% agarose gel containing formamide and then transferred to a GeneScreen Plus membrane (Perkin Elmer). The membrane was fixed and hybridized with α- 32 P-labelled DNA probe made with a High Prime (Roche) at 42 °C overnight in hybridization buffer (50% formamide, 1×SSPE (1×SSPE is 0.18 M NaCl, 10 mM NaH 2 PO 4 and 1 mM EDTA, pH7.7), 4% dextran sulfate, 5×Denhaldt's and 1% SDS). After hybridization, the membrane was washed at 42 °C in 2×SSC containing 0.1% SDS and then subjected to autoradiography. Reverse transcriptase PCR Total RNA was isolated at the different time points as described above and treated with RNase-free DNase I (Promega) at a concentration of 1 unit per mg total RNA in the presence of RNase inhibitor (Roche). RT–PCR was performed using the protocol for the Transcriptor first strand cDNA synthesis kit (Roche), and the primers for four genes were designed to amplify the fragment containing the seven-base sequence cutting site ( Supplementary Table S1 ). PCR was carried out using the primers ( Supplementary Table S1 ). The products were analysed on a 1.2% agarose gel in 1×TBE buffer. Bioinformatics analysis of the cleavage sites for MazF-hw Using Perl programming language for computational analysis, MS2RNA, E . coli 16S and 23S rRNAs and the yeast 18S and 26S rRNAs were analysed for the presence of all possible four-, five- and six-base combinations around the sequence of the sole cleavage site found in MS2 RNA. The genomic ORF sequences of H. walsbyi DSM 16790 from NCBI RefSeq (Accession NC_008212 ) were retrieved and the number of UUACUCA sequences was estimated by using Perl script. For function clustering of each gene, two clusters (clusters of orthologous groups of proteins (COGs) and HaloLex Function class) were used from NCBI and HaloLex database, respectively. COGs were created by comparing protein sequences encoded in complete genomes, representing major phylogenetic lineages. Each COG consists of individual proteins or groups of paralogues from at least 3 lineages and thus corresponds to an ancient conserved domain [23] . HaloLex ( http://www.halolex.mpg.de ) is a comprehensive genome information system for archaea, and the function classes of HaloLex are used to analyse all MazF-hw-sensitive genes [12] . How to cite this article: Yamaguchi, Y. et al . Inhibition of specific gene expression by protein-mediated mRNA interference. Nat. Commun. 3:607 doi: 10.1038/ncomms1621 (2012).